Eliminating the need for anodic gas separation in CO2electroreduction systems via liquid-to-liquid anodic upgrading Electrochemical reduction of CO 2 to multi-carbon products (C 2+ ), when powered using renewable electricity, offers a route to valuable chemicals and fuels. In conventional neutral-media CO 2 -to-C 2+ devices, as much as 70% of input CO 2 crosses the cell and mixes with oxygen produced at the anode. Recovering CO 2 from this stream adds a significant energy penalty. Here we demonstrate that using a liquid-to-liquid anodic process enables the recovery of crossed-over CO 2 via facile gas-liquid separation without additional energy input: the anode tail gas is directly fed into the cathodic input, along with fresh CO 2 feedstock. We report a system exhibiting a low full-cell voltage of 1.9 V and total carbon efficiency of 48%, enabling 262 GJ/ton ethylene, a 46% reduction in energy intensity compared to state-of-art single-stage CO 2 -to-C 2+ devices. The strategy is compatible with today’s highest-efficiency electrolyzers and CO 2 catalysts that function optimally in neutral and alkaline electrolytes. The electrochemical conversion of CO 2 (CO 2 RR) to multi-carbon (C 2+ ) products is a promising approach to reducing net CO 2 emissions [1] . The best existing CO 2 RR flow cell systems [2] , [3] and zero-gap membrane electrode assembly (MEA) systems [4] , [5] , [6] achieve C 2+ Faradaic efficiencies (FEs) of 70% and C 2+ partial current densities of over 1 A cm −2 in flow cells and over 100 mA cm −2 in MEAs. These productivity levels are in a regime of interest with respect to industrial application [7] . Nevertheless, the total energy required for present-day CO 2 -to-C 2+ electrolysis is too high—for example, when targeting ethylene, today’s electrosynthesis systems require fully 8× more energy to produce ethylene than is embodied in the product [8] , [9] . Major energy costs are incurred in the electrolyser and the downstream separation steps (see Methods: Energy assessment and Supplementary note 1 in SI) [7] , [9] . Established approaches to reducing the electrolysis energy requirements include increasing the selectivity for the target product [5] , [6] and incorporating alternative anode reactions [1] , [10] , [11] , [12] , [13] . The major energy and economic penalties associated with downstream separation of CO 2 remain a challenge [14] . Downstream separation is required to isolate products and recover unconverted CO 2 from the product streams and electrolytes [9] . Recovering CO 2 is particularly costly, requiring 25% and 70% of total energy input in the case of neutral and alkaline media CO 2 -to-C 2+ electrolysers, respectively [8] , [15] . Present-day CO 2 RR catalysts operate with highly alkaline local conditions (pH > 12) to promote C 2+ generation at the cathode [2] . However, the carbonate-forming side reaction (CO 2 + OH − → CO 3 2− or HCO 3 − ) is favored under alkaline conditions, consuming the majority of the CO 2 injected [4] , [6] , [15] . Operating with neutral electrolytes (e.g., KHCO 3 ) in a membrane electrode assembly cell mitigates CO 2 loss. However, a significant amount of input CO 2 (~3× more than the fraction that converted to C 2+ ) crosses the anion exchange membrane (AEM) to the anode as carbonate/bicarbonate, combining with the protons generated from the anodic reaction and is converted back to CO 2 (Fig. 1a ) [4] , [15] . Fig. 1: All-liquid anode enabling CO 2 recycling and low energy intensity ethylene. a Mass balance of the electrochemical process in the conventional CO 2 RR-OER electrolysers. b Operating principle of the conventional CO 2 RR-OER electrolysis. F1, F2, F3, and F4 are the CO 2 that: is input, crosses over, is converted to products, and is unreacted, respectively. c Mass balance of the electrochemical process in the CO 2 RR-OOR MEA electrolyser. The MEA-type electrolyser uses a Cu-loaded gas diffusion electrode as the cathode, a Pt/C loaded hydrophilic carbon cloth as the anode, and an anion-exchange membrane (AEM) as the solid-state electrolyte. At the cathode, some CO 2 is electrochemically converted to CO 2 RR products, and a significant fraction of CO 2 is converted to carbonate/bicarbonate due to the high local pH. The carbonate/bicarbonate ions then migrate to the anode through the AEM. An organic precursor is electrochemically oxidized to value-added product(s) in a near-neutral electrolyte and generates protons at the anode. The protons combine with the carbonate/bicarbonate ions, regenerating CO 2 as the only gas-phase product at the anodic product stream. d The operating principle of the CO 2 RR-OOR electrolysis system combines low-energy input and high-carbon utilization in CO 2 -to-C 2+ conversion. The system uses an anolyte composed of KHCO 3 and liquid organic precursors. The cathode chamber is fed with humidified CO 2 . The mass balance table is provided as Table S1 . e Energy intensity of ethylene production in benchmark systems from literature (Neutral MEA [4] ; acidic flow cell [14] ; acidic MEA [21] ) versus this work. Full size image On the anode side, crossover CO 2 combines with O 2 produced via the oxygen evolution reaction (OER) to produce a gas mixture of 60–80% CO 2 and 20–40% O 2 [16] , [17] . This mixture cannot be directly recycled into the cathode because oxygen reduction would dominate at the cathode [18] . As a result, separation of CO 2 is required downstream of the anode, incurring an energy penalty of an added 50–100 GJ per ton of ethylene produced (see Supplementary note 1 )—an energy cost greater than the energy consumption of petrochemical ethylene production (67.5 GJ ton −1 ) [19] . Recent energy and techno-economic assessments demonstrated that this level of separation penalty associated with anodic CO 2 recovery is prohibitive [9] , [15] , [20] . Operating under acidic conditions [14] , [21] , [22] offers one emerging strategy to eliminate CO 2 crossover and the associated anodic separation energy. However, for now at least, this approach incurs high energy costs in the electrolysis step linked to the high full-cell voltage and low C 2+ FE in an acidic environment (Fig. 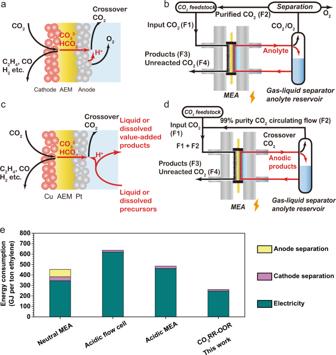Fig. 1: All-liquid anode enabling CO2recycling and low energy intensity ethylene. aMass balance of the electrochemical process in the conventional CO2RR-OER electrolysers.bOperating principle of the conventional CO2RR-OER electrolysis. F1, F2, F3, and F4 are the CO2that: is input, crosses over, is converted to products, and is unreacted, respectively.cMass balance of the electrochemical process in the CO2RR-OOR MEA electrolyser. The MEA-type electrolyser uses a Cu-loaded gas diffusion electrode as the cathode, a Pt/C loaded hydrophilic carbon cloth as the anode, and an anion-exchange membrane (AEM) as the solid-state electrolyte. At the cathode, some CO2is electrochemically converted to CO2RR products, and a significant fraction of CO2is converted to carbonate/bicarbonate due to the high local pH. The carbonate/bicarbonate ions then migrate to the anode through the AEM. An organic precursor is electrochemically oxidized to value-added product(s) in a near-neutral electrolyte and generates protons at the anode. The protons combine with the carbonate/bicarbonate ions, regenerating CO2as the only gas-phase product at the anodic product stream.dThe operating principle of the CO2RR-OOR electrolysis system combines low-energy input and high-carbon utilization in CO2-to-C2+conversion. The system uses an anolyte composed of KHCO3and liquid organic precursors. The cathode chamber is fed with humidified CO2. The mass balance table is provided as TableS1.eEnergy intensity of ethylene production in benchmark systems from literature (Neutral MEA4; acidic flow cell14; acidic MEA21) versus this work. 1e , Table 1 ): today the energy intensity of producing ethylene in acidic CO 2 RR electrolysers is higher than that in conventional AEM-based electrolysers (Fig. 1e , Table 1 ). The further effort needs to be devoted to developing new catalysts and systems for addressing the voltage, selectivity, and stability problems caused by the acidic environment. Table 1 Energy assessment comparison between the state-of-art CO 2 -to-ethylene CO 2 RR devices. Full size table We pursued a strategy that enables the direct recovery of CO 2 from the anodic gas stream without energy penalty. As in prior works, the cathode chamber of the MEA electrolyser is continuously supplied with CO 2 . The anode chamber employs a near-neutral anolyte (e.g., 1 M KHCO 3 ) containing a liquid-phase precursor to be electrochemically oxidized. The AEM separates cathode and anode and provides the locally alkaline conditions favorable for CO 2 RR. In this system, some of the input CO 2 (flow rate: F1 mol s −1 ) crosses over to the anode; some is converted to products (F3); some passes the MEA (F4) with the products. A key feature of the system is the fact that the anode outlet gas can be recirculated (F2) as an inlet gas to the cathode. The carbon efficiency is defined as: [14] 
    Carbon efficiency ( %)=F3/F1× 100 %
 (1) In an ordinary AEM-based, zero-gap CO 2 RR-OER electrolyser (Fig. 1a, b ), a large portion of input carbon (F2, roughly triple to F3 [4] , [6] ) crosses over from the cathode to the anode and combines with the protons from the anodic process to regenerate gaseous CO 2 . Without recirculation, this system shows a carbon efficiency (<30%) close to that of ordinary MEA electrolysers. We noted that if the anodic reaction is designed to be all-liquid in nature— i.e., if it avoids O 2 evolution—then the approach avoids contamination of this CO 2 stream with O 2 . The recovered CO 2 is of high purity (>99%), enabling direct recycling to the cathode (Fig. 1d ), i.e., F1 = F3 + F4 . Such a system breaks the 25% CO 2 utilization limit [15] in AEM-based electrolyzers, avoids the full energy penalty associated with anodic gas separation, and does so without incurring penalties to full-cell voltage or selectivity to ethylene [7] . The approach requires an all-liquid-phase anodic process that produces protons (or consumes hydroxides) and operates in near-neutral media. Candidate anode reactions include water-to-hydrogen peroxide [23] , [24] , chloride-to-hypochlorite [25] , and a wide range of organic oxidation reactions (OORs) [13] , [26] , [27] . However, previously-published catalysts for hydrogen peroxide and hypochlorite production result in gaseous by-products [23] , [24] , [25] . Here we adopt the organic oxidation reaction at the anode. Recent techno-economic analyses [1] , [27] have suggested substituting OER with OOR as an opportunity to reduce full-cell voltage and produce salable products from both sides of the cell. Candidate OOR reactions include the oxidation of glucose [1] , glycerol [1] , furfural [27] , 5-hydroxymethylfurfural [28] , alcohols [10] , [11] , [12] or any other biomass polyols and simple sugars. The coupling of CO 2 RR and the oxidation of organics has been demonstrated in H-cells [10] , [11] , [12] , [28] , [29] , liquid-fed flow cells [30] , gas-fed flow cells [1] , [13] , and MEA electrolysers [31] . Coupling electrochemical CO reduction with OOR has been recently demonstrated in an MEA electrolyser [8] . However, prior systems that employed OOR as an anodic process did not focus on overall carbon efficiency: recent gas-CO 2 -fed CO 2 RR-OOR systems operated in strong alkaline electrolytes (pH > 14) [1] , [13] , [31] , causing a severe energy penalty associated with the regeneration of (bi)carbonate back to alkaline and CO 2 . Glucose is abundant from biomass, with an average market price of $400-500 ton −1 [32] , mainly produced from starch. In 2017, over 5 million tons of glucose were produced in the United States ( https://www.statista.com/statistics/496485/glucose-production-in-the-us/ ). Electrochemical oxidation of glucose produces gluconate, glucuronate, and glucarate (Fig. S1 ) [33] , [34] , and these are feedstocks for the production of biopolymers [35] and pharmaceuticals [36] . Gluconic acid commands a market price of $700–1600/ton [32] , [37] , [38] . The projected market size of gluconic acid is $80 million [39] (2024). Recent techno-economic assessments estimated that [32] , [40] renewable energy-powered electrochemical glucose oxidation reaction (GOR) is economically feasible. GOR outcompetes OER at industrially relevant reaction rates in neutral and near-neutral electrolytes [41] . GOR also offers electrolysis energy savings, with a thermodynamic potential of 0.05 V [1] , significantly lower than that of OER (1.23 V). In this work, we couple the CO 2 RR with the glucose oxidation reaction (GOR) and demonstrate the liquid-phase anodic process strategy. The system shows a low full-cell voltage of 1.9 V and total carbon efficiency of 48%, enabling 262 GJ/ton ethylene, a 46% reduction in energy intensity compared to state-of-art single-stage CO 2 -to-C 2+ devices. Catalyst characterization To perform CO 2 RR on the cathode, we deposited Cu nanoparticles and perfluorosulfonic acid (PFSA) ionomer on a hydrophobic porous polytetrafluoroethylene (PTFE) gas diffusion electrode. The PTFE gas diffusion electrode was pre-sputtered with 200 nm-thick polycrystalline Cu to improve electrical conductivity (see Methods for details). Scanning and transmission electron microscopy (SEM and TEM, respectively) images reveal a surface morphology composed of Cu nanoparticles bonded by several tens of nm-thick PFSA ionomer films (Fig. 2a ). The anode electrode comprised a homogeneous blend of Pt/C nanoparticles and PFSA ionomer on a hydrophilic and highly porous carbon fiber cloth substrate (see Methods for further details). SEM images confirm that the anode is composed of macroporous carbon fibers (Fig. 2b ) that are homogeneously covered by Pt/C nanoparticles and PFSA composites (inset in Fig. 2b ). TEM images in Fig. 2c show that the diameter of Pt nanoparticles is in the range 5–10 nm. Energy-dispersive X-ray spectroscopy (EDS) elemental mapping reveals that Pt is evenly distributed on the surface of C nanoparticles (Fig. 2e and g ). Fig. 2: Electron microscopy characterization of MEA electrolyser catalysts. a Scanning electron microscopy (SEM) and transmission electron microscopy (TEM, inset) images of the cathodic catalyst: Cu nanoparticles/PFSA composite. b SEM images of the anodic catalyst: Pt/C loaded on hydrophilic carbon fibers. c SEM images of the Pt/C catalyst. d – g The scanning transmission electron microscopy image ( d ) and corresponding Energy-dispersive X-ray spectroscopy (EDS) elemental mappings of carbon ( e ), platinum ( f ), and overlap ( g ) for Pt/C catalyst. Full size image Electrochemical characterization of the CO 2 RR-GOR system We conducted linear scan voltammetry (LSV) measurements to investigate the electrochemical response of the CO 2 RR-GOR system with a cathode Cu loading of 0.5 mg cm −2 and an anode Pt loading of 2 mg cm −2 (Fig. 3a and b ). When we did not add glucose to the anolyte (CO 2 RR-OER), the electrolyser delivered a current density of 94 mA cm −2 at a full-cell voltage of 3 V. At 100 mA cm −2 , when we introduced glucose, increasing its concentration in the anolyte from 0.1 to 0.5 M and 1 M, the full-cell voltage decreased from 2.90 to 2.18 V and 2.23 V. The full-cell voltages at glucose concentrations 0.5 M and 1 M are rather close to one another: this we attribute to the electrokinetic limitations of the anode [42] : at 0.5 M, glucose molecules saturate the active sites of the Pt catalyst, and, as a result, increasing the concentration to 1 M does not enable further reduction in the cell voltage. A further increase in the glucose concentration to 2 M increased full-cell voltage, i.e., 2.40 V at 100 mA cm −2 due to the excess coverage of Pt with glucose and oxidation intermediates [43] . We thus adopted 1 M glucose for the performance investigations. Fig. 3: Performance of the CO 2 RR-GOR electrolysis system. The mass loadings on the cathode and anode are Cu: 0.5 mg cm −2 and Pt: 2 mg cm −2 . a , b The linear scan voltammetry (LSV) of the CO 2 RR-GOR electrolysis system with various glucose concentrations (0 M refers to CO 2 RR-OER on a high-surface-area IrO x -Ti catalyst) at 20 o C ( a ) and ( b ) with 1 M glucose at various temperatures. All the profiles were recorded at a scanning rate of 5 mV s −1 immediately after three cycles of voltammetry scanning. c The full-cell potentials of the CO 2 RR-GOR at various temperatures which are measured by applying constant currents. d CO 2 RR FE distributions at 50 o C and a number of different current densities. The liquid FEs are based on the sum of products detected from cathodic + anolyte outlets. e FE distributions of liquid products (measured by NMR and GC) of GOR at various current densities at 50 o C. GOR products were also quantified using HPLC, see Fig. S13 . f The CO 2 and O 2 flow rates (normalized by electrode geometric area) in the anodic gas streams at 50 o C. The simulated CO 2 is assessed by the stoichiometry of generated OH - and transferred electrons, assuming CO 2 is converted to CO 3 2- . g Recovery efficiency and purity of CO 2 at the anodic product stream at various current densities and 50 o C. Recovery efficiency is defined by dividing the CO 2 flow rate from measurement by that from prediction. h The FE distributions of gas products of CO 2 RR at various temperatures and current densities. Full size image Performing LSV and chronopotentiometry measurements, we investigated the voltage-current density dependence at various temperatures (Fig. 3b and c ). Elevating the operating temperature from 20 to 35 o C lowers the full-cell voltage by 0.1–0.3 V in a wide range of current densities from 80 to 160 mA cm −2 (Fig. 3b and c ), attributed to accelerated electrochemical kinetics. A similar full-cell voltage reduction was observed as the operating temperature increased from 35 to 50 o C. Achieving high ethylene FE and low oxygen FE simultaneously Maintaining a low OER FE is critical to ensure high GOR efficiency and sufficient purity of the recovered CO 2 . In the present CO 2 RR-GOR system, we found that the cathodic and anodic catalysts needed to be carefully engineered to enable the CO 2 recovery strategy. In prior studies, typical mass loadings of the cathode Cu (CO 2 RR) and anode Pt (GOR) were 1 mg cm −2 [6] , [44] and 0.5 mg cm −2 [8] . When we used these configurations in our CO 2 RR-GOR system, we obtained high full-cell voltages of >3.4 V when seeking to operate above 100 mA cm −2 , Fig. S5a , showing little advantage over CO 2 RR-OER systems (Fig. S3 ). The high full-cell voltage degraded the selectivity of GOR over OER, leading to an anodic O 2 FE of >8% (Fig. S5b ). Reexamining Pt loading was essential to reduce the full-cell voltage to <2.4 V (Fig. S5a ), and consequently the O 2 FE to <1% (Fig. S5b ) at the current density of 120 mA cm −2 . However, operating at this current density, the CO 2 RR selectivity toward ethylene is ~30% (Fig. S5c, d ), significantly lower than the 40–45% benchmark for Cu [4] , [6] . To achieve this benchmark, the system must run at 200 mA cm −2 (Fig. S5d ) with the full-cell voltage of 3.23 V and O 2 FE of 7% (Fig. S5a, b ). This is not overcome by further increasing Pt loading (Fig. S5a ), as discussed in Fig. S5 . Tuning the Cu loading changes the current density required to maximize the ethylene FE. We, therefore, pair a 0.5 mg cm −2 Cu cathode with a 2 mg cm −2 Pt anode to achieve maximum ethylene FE and low oxygen FE simultaneously at industrial-relevant current densities. When run at 100 mA cm −2 and 50 o C, the CO 2 RR-GOR system provides a full-cell voltage of 1.8 ± 0.1 V, representing a 1.6 V lower voltage than the conventional CO 2 RR-OER system at the same current density and temperature [4] . We attribute this low full-cell voltage to the lower thermodynamic potential of GOR than OER (0.05 vs. 1.23 V) and the anodic catalyst’s high activity toward GOR. Such a low full-cell potential significantly reduces electricity demand (Table 1 ). At 100 mA cm −2 , the system delivers ethylene FEs of 42%, 48%, and 44% at 2 o C, 35 o C, and 50 o C (Figs. S7, 3d , Tables S5 , S6 and S8 ). The Cu-sputtered on the PTFE GDE is unlikely to participate in CO 2 RR: we observed similar performance when spraying Cu nanoparticles onto a hydrophobic carbon paper (Fig. S4 ). We investigated the selectivity of the GOR in a wide range of current densities (from 80 to 160 mA cm −2 ) and operating temperatures (Fig. 3e , Tables S7 and S9 ). With the temperature increasing from 20 to 50 o C, we detected a slight increase in anolyte pH (from pH 7.9 to 8.3, Fig. S10 ), attributable to the lower solubility of CO 2 in warmer anolyte. We detected gluconate as the major GOR product (>49% FE), achieving a plateau of 58% at 140 mA cm −2 . The full analysis of GOR products is shown in Figs. S12 and S13 . The FEs toward oxygen remained <3% at current densities from 80 and 160 mA cm −2 (<1% at 100 mA cm −2 and a full-cell voltage of 1.80 V) owing to the sluggish kinetics of OER (Fig. 3a ). Recycling CO 2 The CO 2 recycling strategy requires a high CO 2 recovery efficiency, in this work defined as: 
    Recovery efficiency=Detected anodic CO_2 flow (mol s^-1)/Theoretical CO_2 crossover (mol s^-1)× 100 %
 (2) 
    Theoretical CO_2 crossover (mol s^-1)=I (A)/F(Cmol^-1)×1/2
 (3) where I refers to the current and F the Faraday constant. Here the CO 2 crossing over to the anode is in the form of carbonate [17] . The experiment suggested that the amount of CO 2 collected at the anode is in good agreement with the stoichiometry of OH - generated and electrons transferred [17] (Fig. 3f ), indicating a CO 2 recovery efficiency approaching 100% (Fig. 3g ). In addition, the anodic CO 2 flow rate is three orders of magnitude larger than that of O 2 (Fig. 3f ), indicating a purity of CO 2 recovered from the anodic gas stream exceeding 99% (Fig. 3g ). This low level of O 2 enables direct recycling of this anode gas stream in the cathode without the need for separation and associated energy costs. Notably, an oxygen fraction of over 1.8% deteriorates the CO 2 RR selectivity, as seen in control studies in Fig. S3 ). Specifically, the cathodic gas product FE distribution (Fig. 3d ) of the CO 2 RR-ORR, with the anodic CO 2 stream directly fed into the cathode, approaches to within 5% absolute the CO 2 RR-OER electrolyser (Fig. S3 ). The control experiments (Figs. S13 , S14 ) and 13 C abundance analysis (Table S4 ) show that >99.8% of the anodic CO 2 is not from the overoxidation of glucose. These experimental observations are in good agreement with the mass balance analysis provided in Fig. 1c . Avoiding the cathode-side CO 2 RR liquid products crossover Ethylene production via CO 2 RR is accompanied by liquid-phase products such as ethanol, acetate, and propanol, much of which crosses the membrane to the anode stream [4] . Cathode-to-anode crossover of liquid products is a challenge in CO 2 RR as these products risk oxidation and dilution in the anolyte. With OOR on the anode side, there is the additional risk that cathode-produced liquids will contaminate the liquid anode product stream and the gaseous CO 2 stream [1] , [27] . When we increased the temperature from 20 to 50 o C, we found that the FEs toward the major gas products of CO 2 RR (C 2 H 4 and CO) increased from 48 to 56% at a constant current density of 100 mA cm −2 (Figs. S4, 3d and h ). This observation agrees with previous studies, attributable to the positive entropy change of the CO 2 RR [45] , [46] . The FE toward the liquid products of CO 2 RR decreased from 24 to 9%—a trend consistent with a previous report [4] . The higher temperature significantly reduced the crossover of ethanol and n-propanol (Fig. S8 ) to the anode side, a finding we assign to the increased rate of evaporation into the cathode gas stream. As a result, the weight ratio of the liquid CO 2 RR products to the GOR target products in the anolyte stream was <1% at 50 o C (Fig. S9 ), in contrast to 1.4% at 35 o C (Fig. S9 ). In light of the evidence that: (i) the total CO 2 RR FE is close to 100% (Fig. 3d , negligible loss due to anode oxidation) and (ii) the ethanol oxidation signal is absent in the CV profiles of the anolyte (Fig. S14 ), we conclude the oxidation of the CO 2 RR liquid products at the anode is insignificant. Thus, operating at modestly elevated temperatures benefits the CO 2 RR-GOR system by reducing full-cell voltage and suppressing the formation and crossover of liquid CO 2 RR products. CO 2 RR-GOR system performance Encouraged by these findings, we explored the carbon efficiency upper limits in the CO 2 RR-GOR system. A widely employed approach [14] , [21] to determine carbon efficiency upper limits is restricting the CO 2 availability at the cathodic stream and measuring the ratio between F3 (CO 2 converted to products) and F1 (CO 2 feeding). The current and FE distributions determine F2 and F3. F1 is regulated to tune the CO 2 availability. In the CO 2 RR-GOR system, F1 = F3 + F4, meaning that F4 needs to be suppressed by lowering F1 to achieve high carbon efficiency. In principle, in a given electrolysis system, the relative values of F1, F2, F3, and F4 are proportional to the electrolyser area. We thus normalize all the flow rates by the electrolyser area in this study to focus in on the intrinsic properties of this system. Decreasing the input CO 2 flow rate increases the carbon efficiency, as is typical in these systems (Table S10 and Fig. 4b ). At an inlet CO 2 flow rate of 0.18 sccm cm −2 (flow rates are normalized by electrode area), the system delivered a total C 2+ FE of ~34% at a constant current density of 100 mA cm −2 and a full-cell voltage of 1.90 V, corresponding to a carbon efficiency of 75% toward all CO 2 RR products (total carbon efficiency, Fig. 4a and b ), exceeding the upper limit of carbon efficiency in neutral media CO 2 RR electrolysers [4] , [6] , [14] . At these conditions the ethylene FE stabilizes at ~26%, corresponding to a CO 2 -to-ethylene carbon efficiency of ~36% (Fig. 4b ). This carbon efficiency is 1.4-fold greater than the theoretical upper limit of 25% in CO 2 -to-ethylene conversion in conventional, neutral-media, AEM-based electrolysers [14] . Restricting the flow rate results in a significant increase in the hydrogen FE (Fig. 4a ), which we and others [4] , [6] , [14] attribute to the mass transfer limitation of CO 2 . GOR maintains consistent selectivity and productivity at the anode, independent from CO 2 availability in the cathodic gas stream (Fig. 4a and Table S11 ). Fig. 4: Performance of the CO 2 RR-GOR system under low CO 2 availability at 50 o C. The mass loadings on the cathode and anode are Cu: 0.5 mg cm −2 and Pt: 2 mg cm −2 . a The FE distributions at various CO 2 input flow rates. The labels are indicated below ( c ). b The CO 2 carbon efficiency for total CO 2 RR and CO 2 -to-C 2 H 4 (mole ratio of the input CO 2 converted to C 2 H 4 ) at various CO 2 input flow rates. c Long-term electrolysis performance with a CO 2 input flow rate of 0.36 sccm cm −2 . The experiments are performed at a current density of 100 mA cm −2 . The flow rate of the CO 2 supplied is normalized by the geometric area of the electrodes. Full size image A trade-off between carbon efficiency and ethylene FE is typical of CO 2 -to-ethylene electrolysis [4] , [6] , [14] (Fig. 4a and b ). A higher carbon efficiency reduces the energy demand for cathode separation, but the accompanying decrease in ethylene FE increases the specific electrolyser energy demand. To reconcile these metrics, we assess the total input energy (electricity, cathode separation, and anode separation per ton of ethylene produced) of various CO 2 RR approaches (see “Methods”) [6] . We find that the CO 2 RR-GOR system achieves the lowest energy consumption of 262 GJ per ton ethylene, and achieves this with the input CO 2 flow rate of 0.36 sccm cm −2 , a total carbon efficiency of 48% toward all CO 2 RR products. Under this condition, the FE toward C 2+ and ethylene are 45% and 32%, respectively (Table 1 ). Compared to state-of-art conventional CO 2 -to-ethylene systems (i.e., MEAs based on AEM and neutral electrolyte), the CO 2 RR-GOR system eliminates the anodic separation energy (>53 GJ per ton ethylene, Supplementary note 1 ). The overall energy intensity of ethylene production is ~46% less than the most energy-efficient prior CO 2 RR systems among neutral and acidic CO 2 -to-ethylene electrolysers (Table 1 ). Stability with high carbon efficiency Stability is a prerequisite for the industrial application of CO 2 RR. However, long-term operation of CO 2 RR with a high carbon efficiency (e.g., CO 2 carbon efficiency >40%) has not been achieved to date. The best CO 2 carbon efficiency achieved for a run duration of 100 h was <4% [6] . We performed extended CO 2 RR under the operating conditions that enable the lowest energy intensity of ethylene production. The CO 2 RR-GOR system achieves stable electrosynthesis of cathodic C 2+ and anodic products for over 80 h at a current density of 100 mA cm −2 , comparable to the stability of conventional MEAs [4] , [5] , [6] . The system maintains an average full-cell voltage of 1.90 ± 0.1 V, an average total C 2+ FE of 42%, and an average carbon efficiency of ~45% toward all CO 2 RR products (Fig. 4c , Table S12 ). Similarly, we detected stable GOR productivity throughout (Fig. 4c , Table S13 ). Notably, this CO 2 -to-C 2+ electrolyser demonstrates high stability while maintaining high carbon efficiency. We demonstrate that pairing CO 2 RR with an all-liquid anodic reaction in neutral media combines high carbon efficiency and low energy input in the electrosynthesis of renewable chemicals and fuels. One key to implementing this strategy is pairing the catalyst mass loadings on the cathode and anode to maximize CO 2 RR product selectivity and minimize anodic OER selectivity simultaneously. The CO 2 that crosses to the anode was recovered from the anodic downstream with a high purity of >99%. By returning CO 2 to the cathodic upstream, this strategy achieves a high CO 2 conversion of up to 75%. The combined system achieves a low full-cell potential of 1.90 V at a current density of 100 mA cm −2 and stable electrosynthesis of C 2+ products for over 80 h while maintaining a high CO 2 conversion of 45%. Accounting for the total electricity and downstream separation energy costs, this method achieves a total energy intensity of 262 GJ per ton of ethylene produced, ~46% lower than that of previous CO 2 RR electrolysers. This work contributes a route to high carbon efficiency in CO 2 RR electrolysis. Materials Potassium bicarbonate (KHCO 3 , 99.7%), D-glucose (99.5%), copper nanoparticles (25 nm), Nafion TM 1100 W (5 wt.% in a mixture of lower aliphatic alcohols and water) and Pt/C (40 wt.% Pt on Vulcan XC72) were purchased from Sigma Aldrich and used as received. Aquivion D79-25BS ionomer was purchased from Fuel Cell Store. Piperion (40 μm) was used as the anion-exchange membrane, purchased from W7Energy and stored in 0.5 M KOH. The water used in this study was 18 MΩ Milli-Q deionized- (DI-) water. Electrodes For the CO 2 RR, we prepared the gas diffusion electrodes (GDEs) by spray-depositing a catalyst ink dispersing 1 mg mL −1 of Cu nanoparticles and 0.25 mg mL −1 of Nafion TM 1100 W in methanol onto a PTFE substrate that pre-sputtered with a 200 nm thick polycrystalline Cu layer. The substrate was prepared by sputtering Cu target, at a rate of 1 Å s −1 onto a piece of PTFE membrane in a Magnetron sputtering system [5] . The mass loading of Cu nanoparticles on the GDE was tuned between 0.5 and 1.0 mg/cm 2 . The GDEs were dried in the air overnight prior to experiments. For the GOR anode electrodes, a commercially available Pt/C was first physically mixed with ionomer (Aquivion D79-25BS) in a glass beaker and then sonicated for 1 h. The resulting catalyst ink was then spray coated on both sides of the hydrophilic carbon cloth until the Pt loading of 0.5–3.2 mg cm −2 was achieved. Characterizations Scanning electron microscopy (SEM) images of cathode and anode were captured by an FEI Quanta FEG 250 environmental SEM. Transition electron microscopy (TEM) images and elemental mappings were acquired by an FEI Titan 80–300 kV TEM microscope. X-ray photoelectron spectra (XPS) of the electrodes were determined by a model 5600, PerkinElmer using a monochromatic aluminum X-ray source. Assembling of the CO 2 RR-GOR system The MEA set (5 cm 2 ) was purchased from Dioxide Materials. A cathode was cut into a 2.5 cm × 2.5 cm piece and placed onto the MEA cathode plate with a flow window with a dimension of 2.23 cm × 2.23 cm. The four edges of the cathode were sealed by copper tapes and then Kapton tapes, and make sure the tapes did not cover the flow window. A Piperion AEM (40 μm, 3 cm × 3 cm) was carefully placed onto the cathode. A gasket with a 2.23 cm × 2.23 cm window was placed on the cathode. The Pt/C loaded carbon cloth anode (2 cm × 2 cm) was placed onto the AEM. Electrochemical measurements All the data in this work were collected with 0.5 mg/cm 2 Cu (cathode) and 2 mg/cm 2 Pt (anode) unless otherwise specified. All the performance metrics were recorded after at least 1000 s of stabilization at a specific condition. The full-cell voltages reported in this work are not iR corrected. All the error bars are presented as standard deviation based on three measurements. The potential cut-off was set to 10 V, and the current applied on the cell was in the range of 0.2–1.0 A. To evaluate the performance of the CO 2 RR-GOR system under different conditions, the cathode side of the MEA was fed with CO 2 flow (0.18–10  sccm cm −2 of electrode area, 10 sccm cm −2 if not specified) that comes from both CO 2 feedstock and anodic gas stream unless specified. The anode side was circulated with a solution containing 1 M KHCO 3 and glucose with various concentrations (0.1–2 M) at 10 mL/min by a peristaltic pump. A gas-tight glass bottle with four in/out channels (gas inlet, gas outlet, liquid inlet and liquid outlet) was used as the anolyte reservoir and gas-liquid separator. In typical CO 2 RR-GOR performance evaluations, the gas inlet channel was sealed, and the gas outlet channel is connected to a ‘Y’ shape tubing connector. Since the anolyte reservoir/gas-liquid separator is gas-tight, the CO 2 pressure between the feedstock stream and anodic stream will eventually be balanced and promote a steady flow rate from both sides. The electrochemical measurements were performed with a potentiostat (Autolab PGSTAT204 with 10 A booster). The auxiliary system for heating the CO 2 RR-OOR electrolyser is shown schematically in Fig. S15 . To evaluate the performance of the CO 2 RR-OER system, the same setup as the CO 2 RR-GOR system was used, except that the anodic gas stream was vented, and the anolyte had no glucose. To evaluate the performance of the HER-GOR system, the cathode was replaced by a Pt/C catalyst spray-coated onto a hydrophobic carbon paper with a loading of 1.0 mg cm −2 . The cathode was fed with 8 sccm cm −2 N 2 to carry out H 2 . Product analysis The CO 2 RR gas products, oxygen, and CO 2 were analyzed by injecting the gas samples into a gas chromatograph (Perkin Elmer Clarus 590) coupled with a thermal conductivity detector (TCD) and a flame ionization detector (FID). The gas chromatograph was equipped with a Molecular Sieve 5 A Capillary Column and a packed Carboxen-1000 Column with argon as the carrier gas. The volumetric gas flow rates in and out of the cell were measured with a bubble column. The FE of a gas product is calculated as follows: 
    FE_i=x_i×VP/RT×n_iF/J
 Where x i is the volume fraction of the gas product i , V is the MEA cathode outlet gas flow rate in L s −1 (measured by a bubble flow meter), P is atmosphere pressure 101.325 kPa, R is the ideal gas constant 8.314 J mol −1 K −1 , T is the room temperature in K, n i is the number of electrons required to produce one molecule of product F is the Faraday Constant 96485 C mol −1 , and J is the total current in A. To analyse the anodic gas stream component, the gas outlet channel of the anolyte reservoir was disconnected from the tubing for circulating to the cathode. A 20 sccm argon flow was input from the ‘gas inlet’ channel of the anolyte reservoir as the carrier gas to promote the accurate analysis of CO 2 and O 2 components in the anode gas. The liquid products from the cathode side of the SC-MEA were collected using a cold trap containing 5 mL 0 o C water. The collected liquid from the cathode side and the anolyte were quantified separately by the proton nuclear magnetic resonance spectroscopy ( 1 H NMR) on an Agilent DD2 500 spectrometer in D 2 O using water suppression mode and dimethyl sulfoxide (DMSO) as the internal standard. Typical 1 H NMR spectra of GOR can be found in Fig. S11 . Fresh anolyte was used for each liquid product quantification plot, and the collection duration was 30~60 minutes. The FE of a liquid product is calculated as follows: 
    FE_i=m_i×n_iF/Jt
 where m i is the quantity of the liquid product i in mole, t is the duration of product collection (1800~3600 seconds). To evaluate the stability of the CO 2 RR-GOR system, the CO 2 RR gas and cathodic product FE were evaluated using the above-mentioned methods. 50 μL of anolyte (the total volume is 10 litres) was periodically (every 15 ~ 20 h) sampled for 1 H NMR analysis. The quantity of the CO 2 RR liquid products that cross over to anolyte and the GOR liquid products in a certain period were deduced from the concentration increment from the beginning to the end of this period. The by-products of the GOR were also measured by high-performance liquid chromatography (UltiMate 3000 HPLC) equipped with an Aminex HPX-87H column (Bio-Rad) and a reflective index detector. The eluent is 0.05 M H 2 SO 4 , and the column was kept at 60 o C. The anodic CO 2 , CO 2 from the cylinder, KHCO 3 and glucose were analyzed for δ 13 C at the Geobiology Isotope Laboratory at the University of Toronto using a Finnigan Gas Bench coupled with a Thermo-Finnigan MAT 253 gas source isotope ratio monitoring mass spectrometer [47] . The Finnigan Gas Bench sample tray was heated to 72 °C and loaded with vials of CO 2 gas samples. Sample vials were first flushed with helium gas. CO 2 samples from the anodic gas stream and cylinder were directly injected into the vials. The KHCO 3 sample reacted with phosphoric acid to release CO 2 . The glucose sample (60~300 μg) reacted with 1 mL oxidant solution (100 mL H 2 O + 4.0 g K 2 S 2 O 8 + 200 mL of 85% H 3 PO 4 ) to release CO 2 [48] . Measured carbon isotopes were compared to the reference materials, CaCO 3 MERCK (in-house standard), IAEA-CO-8, NBS-19 and IAEA-CO-1 (International Atomic Energy Agency Reference Products for Environment and Trade). Carbon isotope data are reported in the standard delta (δ) notation relative to Vienna Pee Dee Belemnite (VPDB). Energy assessment We evaluated the energy consumptions for electrolyser electricity, cathodic separation, and anodic separation in the context of ethylene—the world’s most-produced feedstock. We consider the state-of-the-art CO 2 RR systems from the literature, including neutral MEA electrolysers, acidic flow-cell, and MEA. This consideration is based on the performance metrics, including selectivity, productivity, and full-cell voltage—a combination of them reflects as energy intensity of producing multi-carbon products (i.e., ethylene). The proximity of these performance metrics will help refine the effect of anodic and cathodic separation on the energy requirement for producing ethylene. We summarize the input parameters to the model for all the systems. The majority of these input parameters listed in Table 1 are from literature [9] and this work. Cathodic gas separation was modeled into two steps: (i) pressure swing adsorption to remove CO 2 ; (ii) cryogenic distillation to separate ethylene from hydrogen and CO. We employed one of the most widely used models [20] (i.e., biogas upgrading) for evaluating the energy cost associated with cathode gas separation. The energy assessment on anodic CO 2 /O 2 separation is evaluated in Supplementary note 1 of SI. For acidic flow-cell and MEA electrolysers, we assume no energy cost associated with the anodic separation considering no CO 2 availability at the anodic gas stream [14] . The separation energy of the anodic GOR products is not included in this assessment. 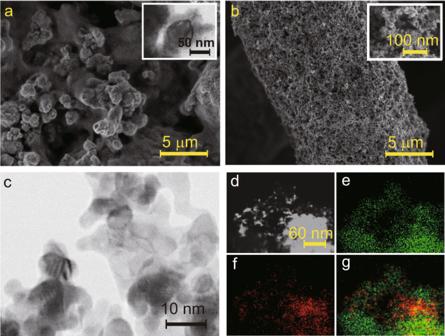Fig. 2: Electron microscopy characterization of MEA electrolyser catalysts. aScanning electron microscopy (SEM) and transmission electron microscopy (TEM, inset) images of the cathodic catalyst: Cu nanoparticles/PFSA composite.bSEM images of the anodic catalyst: Pt/C loaded on hydrophilic carbon fibers.cSEM images of the Pt/C catalyst.d–gThe scanning transmission electron microscopy image (d) and corresponding Energy-dispersive X-ray spectroscopy (EDS) elemental mappings of carbon (e), platinum (f), and overlap (g) for Pt/C catalyst. A previous techno-economic assessment [40] on the electrochemical GOR suggested that the overall process of the electrochemical GOR is economically feasible. 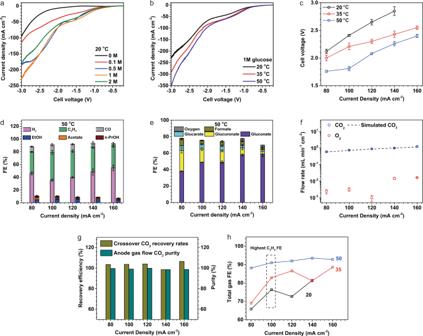Fig. 3: Performance of the CO2RR-GOR electrolysis system. The mass loadings on the cathode and anode are Cu: 0.5 mg cm−2and Pt: 2 mg cm−2. a,bThe linear scan voltammetry (LSV) of the CO2RR-GOR electrolysis system with various glucose concentrations (0 M refers to CO2RR-OER on a high-surface-area IrOx-Ti catalyst) at 20oC (a) and (b) with 1 M glucose at various temperatures. All the profiles were recorded at a scanning rate of 5 mV s−1immediately after three cycles of voltammetry scanning.cThe full-cell potentials of the CO2RR-GOR at various temperatures which are measured by applying constant currents.dCO2RR FE distributions at 50oC and a number of different current densities. The liquid FEs are based on the sum of products detected from cathodic + anolyte outlets.eFE distributions of liquid products (measured by NMR and GC) of GOR at various current densities at 50oC. GOR products were also quantified using HPLC, see Fig.S13.fThe CO2and O2flow rates (normalized by electrode geometric area) in the anodic gas streams at 50oC. The simulated CO2is assessed by the stoichiometry of generated OH-and transferred electrons, assuming CO2is converted to CO32-.gRecovery efficiency and purity of CO2at the anodic product stream at various current densities and 50oC. Recovery efficiency is defined by dividing the CO2flow rate from measurement by that from prediction.hThe FE distributions of gas products of CO2RR at various temperatures and current densities. 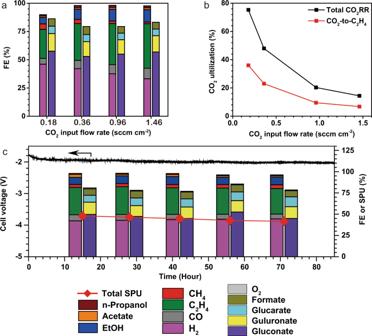Fig. 4: Performance of the CO2RR-GOR system under low CO2availability at 50oC. The mass loadings on the cathode and anode are Cu: 0.5 mg cm−2and Pt: 2 mg cm−2. aThe FE distributions at various CO2input flow rates. The labels are indicated below (c).bThe CO2carbon efficiency for total CO2RR and CO2-to-C2H4(mole ratio of the input CO2converted to C2H4) at various CO2input flow rates.cLong-term electrolysis performance with a CO2input flow rate of 0.36 sccm cm−2. The experiments are performed at a current density of 100 mA cm−2. The flow rate of the CO2supplied is normalized by the geometric area of the electrodes. We, therefore, assume that the energy consumed for anodic GOR product purification can be fully covered by selling the value-add GOR products and does not include it in the comparison between different CO 2 RR devices.